Analysing the relationship between the fields of thermo- and electrocatalysis taking hydrogen peroxide as a case study Currently, >95% of H 2 O 2 is produced by the anthraquinone oxidation process first established in 1939 (Fig. 1a ) [13] . The high capital cost results in large-scale, centralized production where highly concentrated organic working solutions are produced. Subsequently, H 2 O 2 has to be extracted and transported over large distances after which it is diluted again and this energy is often effectively wasted [14] , [15] . Distributed H 2 O 2 manufacture at the point of use is becoming an attractive alternative and would allow production to be integrated into processes permitting (i) minimal time between H 2 O 2 synthesis and use reducing storage requirements, (ii) potential to use stabilizer-free H 2 O 2 for more efficient oxidation processes, (iii) increased raw material security, and (iv) process intensification. Fig. 1: Methods to produce H 2 O 2 Schematic of the anthraquinone process. Schematic of the anthraquinone process ( a ) direct synthesis ( b ), and electrocatalytic method ( c ) to produce H 2 O 2 at the cathode while hydrogen is being oxidized ( d ) Scheme of the mechanism for direct synthesis of H 2 O 2 on Pd proposed by Abate et al. Figures adapted with permission from reference [28] , Springer Nature (2006). e Scheme of the non-Langmuirian proposed mechanism for direct synthesis of H 2 O 2 . f H 2 O 2 concentrations as functions of time during direct synthesis in protic (methanol-black and water-red) or aprotic (dimethyl sulfoxide-green, acetonitrile-blue, and propylene carbonate-magenta) media. g Scheme of the Langmuir mechanism for direct synthesis of H 2 O 2 . Figures adapted with permission from reference [51] , American Chemical Society (2016). Full size image The direct reaction of H 2 and O 2 using thermocatalysis (direct synthesis of hydrogen peroxide, DSHP) is shown in Fig. 1b [16] . One major limitation is the precious metal content of the most efficient Pd and Pt catalysts, or their bi- and trimetallic alloys with Au [17] , [18] , [19] . However, the major limiting factor remains reaction selectivity to prevent water formation by direct combustion or over-hydrogenation and decomposition of H 2 O 2 . Another promising alternative is the electrochemical synthesis by a selective 2-electron oxygen reduction reaction (ORR); which is shown in Fig. 1c [20] . Similar to thermocatalysis, the design of more active and selective catalysts while decreasing the noble metal content remains a challenge. Pd catalysts dominate and the developed approaches to improve selectivity are similar in both fields. These include alloying to exploit electronic effects; site isolation to exploit geometric effects and selective surface blocking to control the concentration and orientation of surface species. Despite diverse reaction paths being possible in thermocatalytic reactions, the Langmuir–Hinshelwood mechanism is often proposed for DSHP, however, the role of charge transfer or changes in oxidation state often are not included in mechanistic steps [21] , [22] , [23] . In general, higher yields of H 2 O 2 can be achieved in acidic conditions or in the presence of protic solvents, however, little consideration is given the role of protons beyond stabilizing the formed H 2 O 2 . Choudhary was among the first to suggest a role of protons in H 2 O 2 formation rather than surface H-atoms by publishing several studies using hydrazine in the absence of H 2 over Pd catalysts and hydroxylamine over Au catalysts [24] , [25] , [26] . This demonstrated that stoichiometric reducing agents can be used in H 2 O 2 production to supply H + /e − , drawing comparisons to electrochemical studies. Seraj et al. explicitly considered H 2 as an electron donor in thermocatalytic nitrite reduction using AuPd catalysts, terminology that is often not considered in the discussion of thermocatalysis [27] . Abate et al . suggested protons hinder the breaking of the O-O bond favoring H 2 O 2 formation over H 2 O (Fig. 1d ), but also implicated protons as mechanistically relevant without consideration of similarities to electrochemical ORR/HOR [28] . An alternative to the Langmuir model has been advanced by Wilson and Flaherty. Studying steady-state H 2 O 2 formation rates over Pd, they found protic media was needed to produce H 2 O 2 and that rates increased with [H + ] drawing a definite dependence on protons in the rate-determining step. Based on this observation, the mechanism proposed is non-Langmuirian (Fig. 1e–g ) where H 2 O 2 is formed by a pathway that involves a water-mediated proton-electron transfer. More recently, Flaherty and co-workers studied the influence of redox mediators such as MeOH in the production of H 2 O 2 [29] . The authors reported that protic solvents generate surface intermediates on Pd that efficiently deliver protons and electrons to catalytic sites. The reaction was reported to consist of spatially decoupled redox reactions with a short-range electron transfer within the metal Pd catalyst. The electrons for the ORR (O 2 + 2H + + 2e − ⇌ H 2 O 2 ) are provided by the HOR (H 2 ⇌ 2H + + 2e − ); thus, the two reactions can occur conceptually at two different sites provided that they are able to transfer electrons and bimetallic samples have shown consistent mechanistic features [18] , [30] . DFT studies on AuPd catalyst materials suggest that protonation of O 2(ads) from water follows a low energy route for both metals; provided a proton shuttle could be set up using two water molecules. This suggests that protonation from solvent molecules represents a reaction pathway with barriers at least as low as the direct hydrogenation from H 2 . The entire process could be considered a sequence of elementary redox processes rather than a purely surface reaction between adsorbed H and O species, consistent with the studies of Ricciardulli et al . on dilute PdAu catalysts with a wide range of compositions [31] . Our own groups demonstrated that single Pd-atom catalysts are able to be highly active and selective in the electrochemical 2e- ORR and HOR and the direct synthesis reaction to produce H 2 O 2 from molecular H 2 and O 2 [32] . Considering these liquid phase reactions as a sequence of elementary redox steps opens new approaches where physically separated half reactions with electrical connectivity can be viewed as fuel cells driven only by chemical potential. Here, the works of Yamanaka et al . can be interpreted as indications of this possibility. The authors described the reaction of H 2 and O 2 gases on physically separated electrodes to avoid mixing H 2 and O 2 [33] , [34] . Here, the HOR on Pt provided a source of protons and electrons that could be directed through an external circuit to drive the ORR. These studies suggest that (i) if electron transfer through the metal is involved, electrochemical studies of thermocatalytic materials can undoubtedly add value to our common knowledge. Furthermore, (ii) the design of new catalysts could be thought of as coupling the most effective structures for the anodic and cathodic half reaction, allowing re-evaluation of materials that have been previously discarded because of activity for only one-half reaction, and (iii) new modes of operation and concepts in material design could be possible with coupled or decoupled sites for each of the ORR and HOR half reactions. Metals such as Au that bind O 2 or O-intermediates weakly tend to be highly selective toward H 2 O 2. However, Au-based catalysts are associated with significant overpotentials (electrochemistry) or low H 2 conversion (direct synthesis) [35] , [36] . Similarly, carbon-based materials are selective to H 2 O 2 in the electrochemical ORR, however, are not active in heterogeneous reactions where H 2 activation is required [37] , [38] , [39] , [40] . Therefore, it seems plausible that catalyst performance could be rationalized by studying the HOR/ORR for thermocatalytic materials electrochemically in isolation. Supporting this hypothesis, Flaherty and co-workers investigated Au-, Pd- and Pt-based catalysts and quantitatively demonstrated the mechanistic similarities between the direct synthesis of H 2 O 2 and synchronous ORR and HOR electrochemistry [41] . The exchange current density, i 0 , can be defined as the rate of the forward and reverse reactions at equilibrium, analogous to a rate constant in thermocatalysis. The equilibrium potential ( E rev ) of each half-cell reaction can be evaluated by thermodynamic considerations while the exchange current density and the Tafel slope account for kinetic contributions. A large I 0 indicates a high level of readiness to proceed with a certain electrochemical reaction. Together with the transfer coefficient (α), Evans diagrams can be derived for a specific catalytic reaction which represents the reaction thermodynamics (potential) and the electrode’s kinetics of a half-cell reaction. These diagrams are common in corrosion science, yet, can be readily extended to coupled redox reactions in catalysis. Evans diagrams for a variety of catalysts for electrocatalytic HOR and ORR are compiled in Fig. 2a including for Pt (black curve) and gold (ochre). The i 0 of HER and ORR for commonly used catalytic materials vary between ~10 −13 A cm −2 (Hg) [42] , [43] , ~10 −6 A cm −2 (Au) [42] , [43] , ~10 −3 A cm −2 (Pd) [42] , [43] , [44] and ~10 −2 A cm −2 (Pt) [44] , [45] . Data concerning non-noble metal candidates was limited due to: (i) poor corrosion resistance under acidic conditions, (ii) unfavorable intermediate adsorption strengths, or (iii) the presence of passivating surface oxides leads to low activity. Fig. 2: Current–voltage curves and complied Evans diagram for HOR and ORR. a Evans diagrams compiled from a variety of catalysts which have been reported as HOR and ORR catalysts. An exhaustive overview of all parameters can be found in Table S1 . Independent current-voltage curves of both half-cell reactions with low ( b ) and high ( c ) HOR and ORR rates as well as one reaction being diffusion limited ( d ) in the framework of the mixed-potential theory. Full size image Initially, without evaluating 2e − vs. 4e − oxygen reduction, we considered the exchange current densities of the 4e − reduction of oxygen to water. Knowing the transfer coefficient allows the exchange current at mixed potentials to be determined in analogy to galvanic processes and is defined as catalytic current density ( j cat ) and catalytic potential ( E cat ). The catalytic potential is the intermediate potential determined by the intersection of the cathodic branch (e.g., ORR) with the anodic branch (e.g., HOR) indicated by the blue line in Fig. 2a shown for Pt. At E cat , the rate of oxygen reduction is equal to the rate of hydrogen oxidation. Thus, if the exchange current density and the Tafel slopes of each half-cell reaction are known, it should be possible to predict the catalytic behavior in thermocatalysis. Conceptually, the higher the catalytic current density between the coupled HOR–ORR redox reactions at relevant conditions, the higher the maximum rate achievable in DSHP reaction (considering overall O 2 reduction to both H 2 O 2 and H 2 O). The reaction rate is therefore limited by the smallest contribution to the ORR/HOR couple. 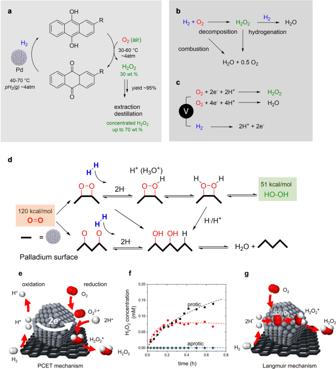Fig. 1: Methods to produce H2O2Schematic of the anthraquinone process. Schematic of the anthraquinone process (a) direct synthesis (b), and electrocatalytic method (c) to produce H2O2at the cathode while hydrogen is being oxidized (d) Scheme of the mechanism for direct synthesis of H2O2on Pd proposed by Abate et al. Figures adapted with permission from reference28, Springer Nature (2006).eScheme of the non-Langmuirian proposed mechanism for direct synthesis of H2O2.fH2O2concentrations as functions of time during direct synthesis in protic (methanol-black and water-red) or aprotic (dimethyl sulfoxide-green, acetonitrile-blue, and propylene carbonate-magenta) media.gScheme of the Langmuir mechanism for direct synthesis of H2O2. Figures adapted with permission from reference51, American Chemical Society (2016). 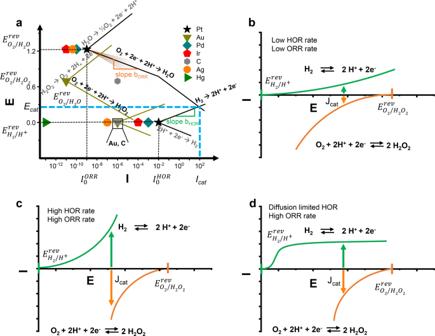Fig. 2: Current–voltage curves and complied Evans diagram for HOR and ORR. aEvans diagrams compiled from a variety of catalysts which have been reported as HOR and ORR catalysts. An exhaustive overview of all parameters can be found in TableS1. Independent current-voltage curves of both half-cell reactions with low (b) and high (c) HOR and ORR rates as well as one reaction being diffusion limited (d) in the framework of the mixed-potential theory. As a benchmark, TOF (h −1 ) and yields (mol kg −1 h −1 ) for the selected heterogeneous catalysts are shown in Supplementary Table 1 . Intriguingly, materials such as Au or Ag possess relatively low catalytic current densities as the half-cell kinetics for the HOR are poor (hypothetically shown in Fig. 2b ) [41] . However, due to low H 2 O 2 residence time and the subsequent hindrance of oxygen adsorption, they tend to demonstrate high selectivity. Despite the relatively low ORR exchange current densities of Au, the reported TOFs are often comparable to metals such as Pt in reactions without acid and halide additives which have larger exchange currents (hypothetically shown in Fig. 2c ) but likely for different reasons (Au—low conversion and high selectivity, Pt—high conversion low selectivity). The reason for this difference can also be qualitatively explained from existing electrochemical studies. Over hydrogenation and H 2 O 2 decomposition takes place due to the high activity for H 2 activation or HOR on Pt compared to Au coupled with strong binding of O-intermediates. The comparison of existing materials hints strongly to the possibility that catalysts can be evaluated separately in half-cells through quick, electrochemical screening and suitable material combinations with electronic connectivity can be combined. However, limitations in comparability between thermo- and electrocatalysis must also be considered. The presumably greatest limitation of comparing both fields lies in their different reaction environments. Most electrochemical approaches are based on using standard conditions for temperature (298.15 K) and pressure (1 bar) in the presence of a conductive and acidic electrolyte with typically low rates of reactant diffusion. High reaction rates in the direct synthesis are also typically limited by reactant solubility in aqueous or alcohol/aqueous based solvent systems. For thermocatalytic systems, working pressures up to 40 bar are common (containing H 2 and O 2 mixtures in a diluent such as N 2 or CO 2 ) and sub-ambient temperatures are often utilized especially in the absence of acid or halide additives to stabilize H 2 O 2 . The exchange current density i 0 also strongly depends on the solution composition adjacent to the electrode’s surface and can be expressed by Eq. 1 . i_0(T,C_O,C_R)=i_0(T^* ,C_O^* ,C_R^* )(C_R/C_R^* )^γ (C_O/C_O^* )^δe^-E_act/RT
 (1) \({i}_{0}\left({{{{{\rm{T}}}}}}^{*},{{{{{\rm{C}}}}}}_{{{{{\rm{O}}}}}}^{* },{{{{{{\rm{C}}}}}}}_{{{{{\rm{R}}}}}}^{* }\right)\) [A \({{{{{{\rm{cm}}}}}}}_{{{{{{\rm{real}}}}}}}^{-2}\) ] as exchange current density at defined reference temperature and reference reactant/product \(({{{{{\rm{C}}}}}}_{{{{{\rm{O}}}}}}^{* },\,{{{{{{\rm{C}}}}}}}_{{{{{\rm{R}}}}}}^{* })\) concentrations, γ, δ as reaction order and E act as activation energy of the exchange current density [46] . From Eq. 1 , the temperature and the surface concentrations can have drastic effects on i 0 . Butler-Volmer kinetics dictate a linear relationship of Tafel slope (b) and temperature, however, a linear dependency of b and T is not always found [47] . The reasons for this have been reported to range from the expansion of the inner region of the double layer with temperature, variable temperature-dependent adsorption of spectator species, structural solvent changes, or to altered solvation spheres around reactant ions [46] . Additionally, diffusion limitation might be depicted as concentration polarization exemplarily shown in Fig. 2d for the HOR. Here, the reaction of H 2 at large overpotentials may cause a depletion of gas and the transport of H 2 to the catalyst’s surface becomes diffusion limited resulting in the shown concentration polarization, effecting directly i cat and E cat . In principle, these limitations could also be measured by electrochemical means. However, in order to allow useful correlation between both fields, interfacial effects in electrocatalysis such as oriented water dipoles, present ions, non-covalent intermediate/water interactions, and the electric field have to be comparably small and Sabatier’s principle (binding intermediates not too strongly and not too weakly) dominates the reaction mechanism. This is often the case as shown by modeling electrochemical processes by conducting gas-phase calculations on well-defined catalytic surfaces [48] , [49] , [50] . Overall, comparing both fields, the thermo- and electrocatalytic H 2 O 2 production reveal many similarities. For both reactions, the catalyst selection narrows down to similar materials, mainly Pd and Pt-based materials. Intriguingly, more materials for the electrocatalytic ORR have been reported that do not appear in the thermocatalytic synthesis of H 2 O 2 . The reason might lie in a non-Langmuirian reaction mechanism where spatially decoupled redox reactions take place. Specifically, the ORR acts as electron sink provided for the hydrogen oxidation reaction when both are electronically connected. These observations are supported by the compilation of potential–current density diagrams that can be used to bridge the gap between both fields. Moreover, the selection of catalyst material is generally dictated by activity considerations only, while strategies to increase the selectivity are often lacking. Further enhancement of the overall performance will greatly rely on the joint optimization of both catalytic properties, eventually guided by the investigations of half-reactions via electrochemical methods. In general, this approach of combining know-how from thermo- and electrocatalysis that has been laid out for the example of H 2 O 2 synthesis can be adapted to a wide range of reactions including oxidation and reduction processes at interfaces. Developments along this path can be mutually beneficial, leading to more efficient chemical technologies and novel applications.